Coulombic self-ordering upon charging a large-capacity layered cathode material for rechargeable batteries Lithium- and sodium-rich layered transition-metal oxides have recently been attracting significant interest because of their large capacity achieved by additional oxygen-redox reactions. However, layered transition-metal oxides exhibit structural degradation such as cation migration, layer exfoliation or cracks upon deep charge, which is a major obstacle to achieve higher energy-density batteries. Here we demonstrate a self-repairing phenomenon of stacking faults upon desodiation from an oxygen-redox layered oxide Na 2 RuO 3 , realizing much better reversibility of the electrode reaction. The phase transformations upon charging A 2 MO 3 (A: alkali metal) can be dominated by three-dimensional Coulombic attractive interactions driven by the existence of ordered alkali-metal vacancies, leading to counterintuitive self-repairing of stacking faults and progressive ordering upon charging. The cooperatively ordered vacancy in lithium-/sodium-rich layered transition-metal oxides is shown to play an essential role, not only in generating the electro-active nonbonding 2 p orbital of neighbouring oxygen but also in stabilizing the phase transformation for highly reversible oxygen-redox reactions. The discovery of intercalation chemistry in layered transition-metal oxides AMO 2 (A=Li, Na and M=transition metal) [1] , [2] in the early 1980s has led to the commercialization of lithium-ion batteries [3] . Tremendous effort has since been devoted to understanding how alkali-metal ions reversibly (de)intercalate in AMO 2 because this is essential to exploit their large theoretical capacities (~275 mAh g −1 for LiCoO 2 and ~235 mAh g −1 for NaCoO 2 , respectively). It is now well understood that, at the early stage of A + deintercalation, A x MO 2 (0.4 < x < 1.0) exhibit an increase of their interlayer distance because the depletion of screening A + layers enhances the effective Coulombic repulsion between oxide ions of adjacent MO 2 layers [4] , [5] , [6] , [7] , [8] . At the late stage of A + deintercalation (0.0 < x < 0.4), high-valent M increases the covalency of M − O bonds, and thus decreases the negative charge on oxide ions. In this situation, O − O van der Waals attraction forces are not sufficient to maintain the layered structure, and the large volume variations induced at the end of charge often initiate crack formation and delamination/exfoliation [8] , [9] , [10] . Furthermore, the lack of alkali ions in the interlayer space leads to structural degradation with migration of transition-metal ions to neighboring tetrahedral sites [11] , [12] , [13] . This established knowledge on the intercalation chemistry of A x MO 2 explains the practical limit of their reversible capacity (approximately for 0.4 < x < 1.0, i.e., 170 mAh g −1 for A = Li and 140 mAh g −1 for A = Na). Therefore, the control of the competing Coulombic and van der Waals forces in layered transition-metal oxides is of great importance to achieve a large reversible capacity. Layered A -excess transition-metal oxides (A 1+ y M 1− y O 2 or A 1 [A y M 1− y ]O 2 ) are recent major targets to increase the cathode capacity by virtue of additional oxygen-redox reactions. Li 2 MnO 3 -LiMO 2 solid solutions have been reported to deliver large capacities over 200 mAh g −1 [14] , [15] , [16] , and have more recently been followed by Li 2 MO 3 (M = Ru [17] , Ir [18] , RuSn [17] , and RuMn [19] ) and Na 2 MO 3 (M = Ru [20] , [21] , RuSn [21] , and Ir [22] ), all delivering large capacities exceeding that of solely M redox. Although the changes in the electronic state during the additional oxygen-redox reactions have been intensively investigated, less attention has been paid to the essential interaction dominating the phase transformation during the charge/discharge processes, presumably because most oxygen-redox electrodes exhibit severe structural degradation (i.e., oxygen-gas evolution, cation migration) at the initial charge [16] , [17] , [23] , [24] . However, the extra A + are expected to play a crucial role in the structural transformation during the charge/discharge processes. For example, the depletion of screening A + layers upon charging can be compensated by the A + supplied  from the [A y M 1− y ]O 2 layers [18] , [20] , [22] . Moreover, A + (or vacancy after deintercalation) in the [A y M 1− y ]O 2 layers is expected to modulate the balance of competing Coulombic/van der Waals forces, and hence largely influence the intercalation chemistry. We have recently studied the structure and electrochemistry of O3-Na 2 RuO 3 (or Na[Na 1/3 Ru 2/3 ]O 2 ), where [Na 1/3 Ru 2/3 ]O 2 layers have a honeycomb-type ordered arrangement of Na and Ru [20] , [25] . According to the classification of layered oxides, O3 denotes a structure where Na + ions occupy octahedral interlayer sites and the stacking of oxide ions is ABCABC (Supplementary Fig. 1) [26] . Importantly, in contrast to most oxygen-redox electrodes, O3-Na 2 RuO 3 exhibits highly reversible (de)sodiation without structural degradation but rather exhibits progressive structural ordering upon charging, which provides an opportunity for not only detailed structural investigation as a model system but also for essential strategies toward much larger reversible capacity. In this work, synchrotron X-ray diffraction coupled with planar-defect refinement analyses are applied to honeycomb ordered Na x RuO 3 phases ( x = 2, 1, and 1/2), revealing a self-repairing phenomenon of stacking faults upon charging, which significantly stabilizes the reversible large capacity operation. Driving force of the 3D self-ordering is strong long-range cooperative Coulombic interactions between MO 3 slabs intermediated by ordered vacancies. Stacking faults in Na 2 RuO 3 O3-Na 2 RuO 3 was synthesized by decomposing Na 2 RuO 4 at 850 °C for 12 h under Ar atmosphere [20] , [25] . 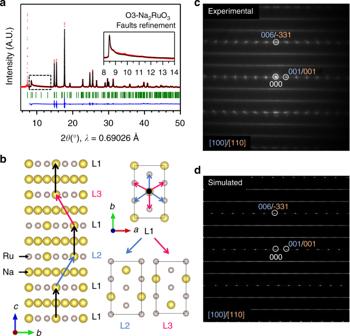Fig. 1 Stacking faults in Na2RuO3.aObserved and calculated (FAULTS refinement) synchrotron XRD patterns of O3-Na2RuO3(pristine state). Observed data, the calculated pattern, and the difference between observed and calculated data are shown as plus sign (red), solid line (black) and continuous line (blue), respectively. The positions of Bragg reflections are indicated by vertical tick marks (green). The first diffraction peak has been excluded from the refinement due to important asymmetry that FAULTS does not take into account. The insert is a zoom of the initial superstructure peaks (Warren fall).bRepresentation of the stacking faults in O3-Na2RuO3, using the FAULTS unit cell described in the text.c,dExperimental and simulated SAED pattern along the [100] (= <[110]C2/m>) direction, respectively Figure 1 a shows the experimental and calculated synchrotron XRD patterns of O3-Na 2 RuO 3 , in which the most of intense diffraction peaks can be fitted by the usual rhombohedral lattice of O3-AMO 2 layered oxides [20] . However, the main difficulty hindering an accurate pattern fit lies in the broad nature of some diffraction peaks and diffuse scatterings, which are highlighted by the dashed rectangle in Fig. 1 a. Such broadening is typically observed for A 2 MO 3 with honeycomb ordered [A 1/3 M 2/3 ]O 2 layers, and arises from stacking disorder. These stacking faults can be described by an occasional shift of the [A 1/3 M 2/3 ]O 2 layers perpendicularly to the stacking direction. In fact, in layered materials, the crystal grows perpendicularly to the layer plane. When a nucleation starts in a wrong position, a stacking fault appears while the oxygen packing remains ideal. As a result, the honeycomb ordering of the [A 1/3 M 2/3 ]O 2 layers is maintained but the honeycomb stacking deviates from the ideal sequence (Fig. 1 b), which causes the peculiar asymmetric peak broadening (Warren fall) observed in Fig. 1 a as well as the diffuse streaks on the selected area electron diffraction (SAED) pattern along the [100]−<110> C 2/ m direction (Fig. 1c). Fig. 1 Stacking faults in Na 2 RuO 3 . a Observed and calculated (FAULTS refinement) synchrotron XRD patterns of O3-Na 2 RuO 3 (pristine state). Observed data, the calculated pattern, and the difference between observed and calculated data are shown as plus sign (red), solid line (black) and continuous line (blue), respectively. The positions of Bragg reflections are indicated by vertical tick marks (green). The first diffraction peak has been excluded from the refinement due to important asymmetry that FAULTS does not take into account. The insert is a zoom of the initial superstructure peaks (Warren fall). b Representation of the stacking faults in O3-Na 2 RuO 3 , using the FAULTS unit cell described in the text. c , d Experimental and simulated SAED pattern along the [100] (= <[110] C 2 / m >) direction, respectively Full size image To refine the powder diffraction data for the structure containing stacking faults, a FAULTS analysis, which allows the incorporation of the occurrence probabilities of possible stackings, was conducted [27] . As shown in Fig. 1 a (Supplementary Tables 1 and 2 ), the FAULTS analysis provides a satisfactory description of the superstructure peaks and indicates the occurrence of ~40% stacking faults between the [Na 1/3 Ru 2/3 ]O 2 layers in pristine O3-Na 2 RuO 3 . This result is further supported by the FAULTS-simulated SAED pattern that well reproduces the diffuse streaks observed in the experimental SAED pattern (Fig. 1d). After evaluation of the stacking faults in pristine O3-Na 2 RuO 3 , we studied the structural evolution of Na x RuO 3 during the first charge and discharge using in situ XRD. 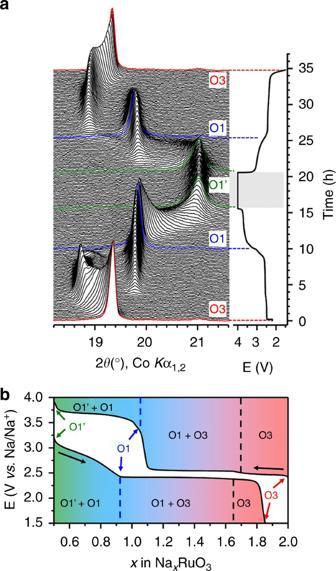Fig. 2 Structural evolution upon charging/discharging Na2RuO3.aXRD patterns recorded in situ during the first cycle of Na2RuO3with the corresponding cycling curve. The dashed area corresponds to a potentiostatic break whose aim was to ensure the equilibrium state at 4.0 V before discharging the cell.bPhase diagram as determined from the in situ experiment as a function of the sodium content Figure 2 shows that the phase transformation of Na x RuO 3 involves three main phases: O3-Na x RuO 3 , O1-Na 1 RuO 3 , and O1′-Na 1/2 RuO 3 . (De)sodiation at 2.7 V vs. Na/Na + (1.0< x <2.0) mainly proceeds through a two-phase process between O3-Na x RuO 3 and O1-Na 1 RuO 3 . As reported previously, O1-Na 1 RuO 3 has an ilmenite-type structure (ABAB oxide-ions stacking and Na + ions in interlayer octahedral sites) where the honeycomb ordered [Ru 2/3 □ 1/3 ]O 2 and [Na 2/3 □ 1/3 ]O 2 layers (□: Na + vacancy) stack alternatively (Supplementary Fig. 2) [20] . At the second charging plateau, a new phase (O1′-Na 1/2 RuO 3 ) with a shorter interlayer distance (4.91 Å vs. 5.21 Å for O1-Na 1 RuO 3 ) appears at the expense of the O1 phase. Its structure was determined from the synchrotron XRD pattern of an electrochemically deintercalated sample, whose Rietveld refinement is presented in Supplementary Fig. 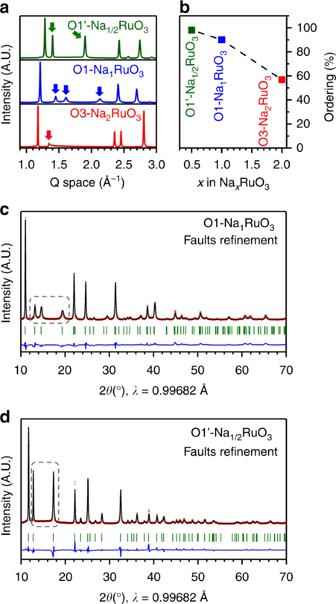Fig. 3 Progressive stacking-fault-depression (self-ordering) upon charging Na2RuO3.aSynchrotron XRD patterns of O3-Na2RuO3, O1-Na1RuO3and O1′-Na1/2RuO3. Arrows indicate the most intense superstructure peaks.bEvolution of the ordered stacking (absence of stacking faults) as a function of the Na content. The error bars are smaller than the mark size.c,dObserved and calculated (FAULTS refinement) synchrotron XRD patterns of O1-Na1RuO3and O1′-Na1/2RuO3, respectively. Red crosses: experimental, black line: calculated, blue line: difference plot and green bars: Bragg positions in the R\(\bar{3}\):h and P\(\bar{3}\)1mspace groups for O1-Na1RuO3and O1′-Na1/2RuO3, respectively. The dashed rectangles indicate the most intense superstructure peaks 3 and Supplementary Table 3 . The diffraction peaks are successfully indexed in a hexagonal lattice with P \(\bar{3}\) 1 m symmetry with a = 5.1876(9) Å and c = 4.906(1) Å. As the oxide-ion stacking sequence is ABAB and Na + occupies an octahedral site, we will refer to this phase as O1′-Na 1/2 RuO 3 , where the alternate stacking of the honeycomb ordered [Ru 2/3 □ 1/3 ]O 2 and [Na 1/3 □ 2/3 ]O 2 layers is maintained. Then, the difference between the O1 and O1′ structures lies in the Na content and on the respective stacking of the [Ru 2/3 □ 1/3 ]O 2 layers, which are shifted from one another in O1-Na 1 RuO 3 while directly stacked in O1′-Na 1/2 RuO 3 (Supplementary Figs. 2 and 3 ). It is noteworthy that the superstructure peaks highlighted by the arrows in Fig. 3a exhibit remarkable sharpening upon charging. This suggests that stacking faults tend to disappear, assisted by the adjustable layer gliding involved in the O3→O1′ transition. 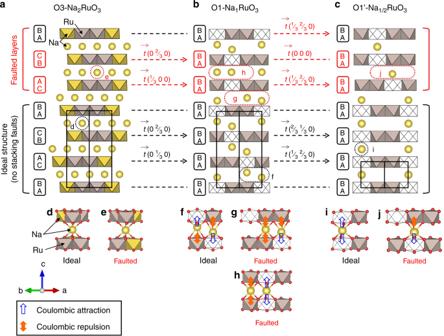Fig. 4 Coulombic forces and resultant stacking–fault–depression (self-ordering) in Na2−xRuO3. Structural representation and projected stacking sequences of the Ru atoms ofaO3-Na2RuO3,bO1-Na1RuO3andcO1′-Na1/2RuO3. The monoclinic cell of O3-Na2RuO3has been converted to a pseudo-hexagonal supercell (black lines) for comparison. The transition vectors in the hexagonal supercell from one [Ru2/3Na1/3]O2or [Ru2/3□1/3O2] layer to another are indicated with respect to the pseudo-hexagonal or hexagonal cells. Note that the transition vectors assigned to faulted layers are a few examples out of many possibilities listed in Supplementary Figs. 5 and 6.d‒jComparison of the Na environments in ideal and faulted stacking highlighted with dashed circles in the structures shown ina‒c The FAULTS refinements (Fig. 3 c, d and Supplementary Tables 4 – 6 ) indicate that the occurrence probability of stacking faults indeed decreases from 40% in O3-Na 2 RuO 3 to 10% (O1-Na 1 RuO 3 ) and then to 2% (O1′-Na 1/2 RuO 3 ) (Fig. 3 b). Therefore, Na + deintercalation (charging) from Na 2 RuO 3 involves a self-reorganization process that significantly diminishes the initial amount of stacking faults. Importantly, the stacking faults are reformed after discharging, making this ordering/faulting process reversible, even after several cycles (Supplementary Figs. 4 and 5). Fig. 2 Structural evolution upon charging/discharging Na 2 RuO 3 . a XRD patterns recorded in situ during the first cycle of Na 2 RuO 3 with the corresponding cycling curve. The dashed area corresponds to a potentiostatic break whose aim was to ensure the equilibrium state at 4.0 V before discharging the cell. b Phase diagram as determined from the in situ experiment as a function of the sodium content Full size image Fig. 3 Progressive stacking-fault-depression (self-ordering) upon charging Na 2 RuO 3 . a Synchrotron XRD patterns of O3-Na 2 RuO 3 , O1-Na 1 RuO 3 and O1′-Na 1/2 RuO 3 . Arrows indicate the most intense superstructure peaks. b Evolution of the ordered stacking (absence of stacking faults) as a function of the Na content. The error bars are smaller than the mark size. c , d Observed and calculated (FAULTS refinement) synchrotron XRD patterns of O1-Na 1 RuO 3 and O1′-Na 1/2 RuO 3 , respectively. Red crosses: experimental, black line: calculated, blue line: difference plot and green bars: Bragg positions in the R \(\bar{3}\) :h and P \(\bar{3}\) 1 m space groups for O1-Na 1 RuO 3 and O1′-Na 1/2 RuO 3 , respectively. The dashed rectangles indicate the most intense superstructure peaks Full size image Self-ordering of stacking faults upon charging Na 2 RuO 3 Based on the complete knowledge of the structural evolution from O3-Na 2 RuO 3 to O1-Na 1 RuO 3 , and then to O1′-Na 1/2 RuO 3 , let us now consider the Coulombic origin of the consolidation on the phase transformation with the effect of gliding vectors t → of the [Ru 2/3 Na 1/3 ]O 2 (or [Ru 2/3 □ 1/3 ]O 2 ) layers (Fig. 4 a–c). Note that the vectors are given in the pseudo-hexagonal cell (O3-Na 2 RuO 3 ) or in the hexagonal cells (O1-Na 1 RuO 3 and O1′-Na 1/2 RuO 3 ; Supplementary Table 7 ). In O3-Na 2 RuO 3 (Fig. 4 a), the NaO 6 octahedron in Na layers shares edges with two NaO 6 and four RuO 6 octahedra in the adjacent [Ru 2/3 Na 1/3 ]O 2 layers (Fig. 4 d). As the stacking faults only impact the stacking of the [Ru 2/3 Na 1/3 ]O 2 layers, the Na + ions in the Na layer have the same local environment (Fig. 4 e) and it can be considered that a different stacking is equally probable in O3-Na 2 RuO 3 . However, in O1-Na 1 RuO 3 consisting of honeycomb ordered [Ru 2/3 □ 1/3 ]O 2 and [Na 2/3 □ 1/3 ]O 2 layers with the ABAB oxygen packing (Fig. 4 b), all the octahedral positions in the slab share faces with the octahedral positions of the interslab space (Supplementary Fig. 6 ). As a result, the gliding vectors t → that shift each layer of O3-Na 2 RuO 3 to the ones of O1-Na 1 RuO 3 are ideally adjusted to set each NaO 6 octahedron in the [Na 2/3 □ 1/3 ] layers to share faces with a □O 6 octahedron and a RuO 6 octahedron in the adjacent [Ru 2/3 □ 1/3 ]O 2 layers (Fig. 4 f and Supplementary Fig. 7 ). The stronger attraction of the oxygen atoms surrounding a vacancy on the Na + ion (later referred to as Na + −□ Coulombic attraction for simplicity) and the Na + −Ru 5+ Coulombic repulsion cooperatively displace the Na + ion toward □ [20] . When assuming the hypothetical stacking faults (Fig. 4 g, h), one of two NaO 6 octahedra is trapped between two RuO 6 octahedra, where strong Ru 5+ −Na + −Ru 5+ Coulombic repulsions make the faulted structural option unfavorable. Consequently, during the O3 to O1 transformation, slab gliding tends to occur in a way which minimizes the Coulombic energy and as a consequence removes the stacking faults, as described in Fig. 4 and Supplementary Fig. 7 . Owing to the three-directional gliding possibilities, most of the stacking faults disappear during the transformation. However, the NaO 6 octahedron can occasionally be stabilized by the local □−Na + −□ Coulombic attraction (Fig. 4 h), and some stacking faults may remain in O1-Na 1 RuO 3 . Fig. 4 Coulombic forces and resultant stacking–fault–depression (self-ordering) in Na 2− x RuO 3 . Structural representation and projected stacking sequences of the Ru atoms of a O3-Na 2 RuO 3 , b O1-Na 1 RuO 3 and c O1′-Na 1/2 RuO 3 . The monoclinic cell of O3-Na 2 RuO 3 has been converted to a pseudo-hexagonal supercell (black lines) for comparison. The transition vectors in the hexagonal supercell from one [Ru 2/3 Na 1/3 ]O 2 or [Ru 2/3 □ 1/3 O 2 ] layer to another are indicated with respect to the pseudo-hexagonal or hexagonal cells. Note that the transition vectors assigned to faulted layers are a few examples out of many possibilities listed in Supplementary Figs. 5 and 6. d ‒ j Comparison of the Na environments in ideal and faulted stacking highlighted with dashed circles in the structures shown in a ‒ c Full size image On the other hand, in O1′-Na 1/2 RuO 3 (Fig. 4 c and Supplementary Fig. 3 b), which consists of honeycomb ordered alternating [Ru 2/3 □ 1/3 ]O 2 and [Na 1/3 □ 2/3 ] layers, the NaO 6 octahedron shares faces with two □O 6 octahedra in the adjacent [Ru 2/3 □ 1/3 ]O 2 layers (Fig. 4c , i). Again with hypothetical stacking faults resulting from t → different from the ideal ones shown in Supplementary Fig. 8 , the NaO 6 octahedron in the [Na 1/3 □ 2/3 ] layer shares faces with □O 6 and RuO 6 octahedra, and the local Na + -Ru 5+ Coulombic repulsion prohibits the formation of the faulted structure (Fig. 4 j). Therefore, the amount of the stacking faults in Na x RuO 3 (1/2 ≤ x ≤ 2) continuously diminishes as desodiation proceeds, because the ordered stacking sequences become electrostatically more favorable. As discussed above, no peculiar local environment is stabilized in O3-Na 2 RuO 3 , which allows for stacking faults reformation upon sodiation (Supplementary Figs. 4 and 5). The aforementioned importance of the attractive A + −□ and repulsive A + −M 5+ Coulombic interactions can lead to more general discussions on the phase stability of A 2 MO 3 and AMO 2 upon charging. 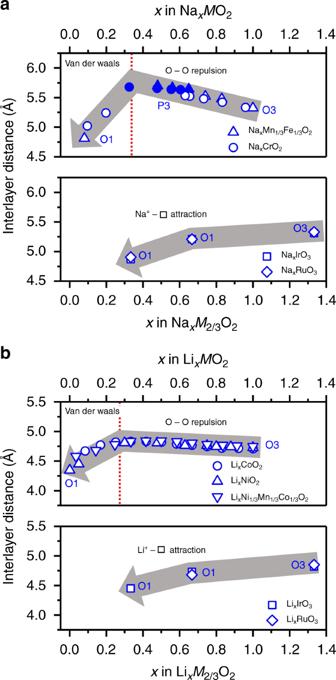Fig. 5 Overviewing dominant forces for phase transformation during A+de-intercalation from AMO2and A2MO3. Comparison of the general trends in interlayer distance evolution betweenaNaxMO2(M = Cr28and Fe2/3Mn1/38) and Na2MO3(M = Ru (this study) and Ir22) andbLixMO2(M = Co4, Ni6and Ni1/3Mn1/3Co1/37) and LixMO3(M = Ru17and Ir18) Figure 5a shows the experimental evolution of the interlayer distance upon charging various Na x MO 2 (M = 3d) [8] , [28] and Na 2 MO 3 (M = 4d, 5d) [22] compounds as a function of the sodium content. Figure 5b shows the similar plots for the lithium analogs, LiMO 2 and Li 2 MO 3 [4] , [6] , [7] , [17] , [18] . It is noteworthy that all AMO 2 (A = Li, Na and M = 3d) and all A 2 MO 3 (A = Li, Na and M = 4d, 5d) respectively follow the same tendencies. Fig. 5 Overviewing dominant forces for phase transformation during A + de-intercalation from AMO 2 and A 2 MO 3 . Comparison of the general trends in interlayer distance evolution between a Na x MO 2 (M = Cr 28 and Fe 2/3 Mn 1/3 8 ) and Na 2 MO 3 (M = Ru (this study) and Ir 22 ) and b Li x MO 2 (M = Co 4 , Ni 6 and Ni 1/3 Mn 1/3 Co 1/3 7 ) and Li x MO 3 (M = Ru 17 and Ir 18 ) Full size image As mentioned in the introduction, the phase transformation of A x MO 2 is dominated by the competing O−O Coulombic repulsion (0.4 < x < 1.0) and van der Waals attraction (0 < x < 0.4) between adjacent MO 2 layers [4] , [5] , [6] , [7] , [8] , which initiates the increase of the interlayer distance (0.4 < x < 1.0) followed by its abrupt decrease upon deeper charging (0 < x < 0.4). Structural evolution in the “Coulombic domain” with large A + content (0.4 < x < 1.0) are highly reversible and is the basis of commercial positive electrode materials such as LiCoO 2 and Li[Ni 1- y - z Mn y Co z ]O 2 , while the “van der Waals domain” with smaller A + content (0 < x < 0.4) marks the limit of reversibility of many practical layered oxides as a result of cation migration, spinel transformation, crack formation, and delamination/exfoliation [8] , [9] , [10] , [11] , [12] , [13] . On the contrary, the highly ordered nature of the [Ru 2/3 □ 1/3 ]O 2 layers of A x MO 3 (M = Ru or Ir) triggers a progressive gain in A + −□ Coulombic energy upon A + extraction as the remaining A + ions cooperatively act as robust pillars between adjacent [Ru 2/3 □ 1/3 ]O 2 layers to prevent structural collapse. The slight decrease of the interlayer distance is driven by Coulombic A + −□ attractive forces which are strong enough to induce the slab glidings, O3 → O1 → O1′, forming a more-ordered structure upon charging. It is this situation that realizes reversible charge–discharge reactions in ordered A 2 MO 3 over a wide compositional domain of the guest ion A + . In summary, we identified a spontaneous reorganization of the stacking faults in Na x RuO 3 , a model material to understand oxygen-redox reactions in layered oxides for large-capacity battery electrodes. In particular, the progressive ordering upon charging process is a general phenomenon to A 2 MO 3 (A = Li, Na and M = 4d, 5d) materials and is induced by the cooperative effect of maximizing the A + −□ Coulombic attraction and minimizing the A + −M 5+ Coulombic repulsion, which significantly enlarges the reversible operation range of layered oxides. Complementarily to our previous work, in addition to generate redox-active “orphaned” nonbonding oxygen 2 p orbitals to “activate” additional oxygen-redox reactions, honeycomb ordering of M and □ contribute to “stabilizing” reversible phase transformation. In this regard, the importance of the overall material design that includes ordered vacancies with its neutral charge to attract alkali cations was highlighted. By establishing proper ways to control the stacking faults [29] , [30] , [31] or vacancies [32] , the concept of progressive ordering upon charging may be extended to stabilize other related compounds [33] . Synthesis of Na 2 RuO 3 Na 2 RuO 3 was prepared according to the literature [25] . First, Na 2 RuO 4 is prepared by mixing stoichiometric amounts of Na 2 O 2 (Sigma-Aldrich) and RuO 2 (Kanto chemicals). Pellets are then made and introduced in a tubular furnace to be annealed at 650 °C for 12 h under O 2 atmosphere. After the synthesis, Na 2 RuO 4 is grinded and shaped into pellets again to be thermally decomposed into Na 2 RuO 3 at 850 °C for 12 h under Ar atmosphere. After cooling down to room temperature, the sample is introduced in an Ar filled glovebox. Characterization The synchrotron XRD patterns were recorded at Aichi Synchrotron Radiation Center (Aichi-SR, O3-Na 2 RuO 3 ), and Photon Factory at High Energy Accelerator Research organization (KEK-PF, BL-8B) or SPring-8 (O1-Na 1 RuO 3 and O1′-Na 1/2 RuO 3 , beamline 02B2). All samples were protected from air exposure during the measurement. Rietveld refinement was performed using Jana2006 [34] . Analyses of the stacking faults in the materials were carried out using the FAULTS software [27] . The crystal structures were drawn using VESTA [35] . Selected Area Electron Diffraction (SAED) patterns were recorded using an electron microscope (HF-3000S; Hitachi Ltd. and Titan Cubed; FEI Co.) operated at 300 kV. The camera length for SAED was calibrated with a Si crystal. Electrochemistry Electrochemical measurements were carried out in Na 2 RuO 3 /electrolyte/Na half-cells assembled in CR2032 type coin cells. The electrolyte was 1 mol/L NaPF 6 in EC:DEC (1:1) purchased from Chameleon Reagent. Positive electrodes were prepared by coating a slurry made of active material (80 wt%) mixed with acetylene black (10 wt%) and polyvinylidene (10 wt%) in NMP onto Al foil. Sixteen-mm-diameter electrodes were cut after drying for one night under vacuum at 120 °C. The positive and negative electrodes were separated by a layer of Whatman glass fiber separator soaked with electrolyte. The galvanostatic curve was recorded and controlled using a TOSCAT-3100 battery tester. The charge/discharge rate was C/10 which corresponds to the (de)intercalation of 1 Na + per Na x RuO 3 in 10 hours. The O1-Na 1 RuO 3 and O1′-Na 1/2 RuO 3 samples were prepared by cycling sintered pellets (diameter 10 mm, weight ≈10–15 mg) of O3-Na 2 RuO 3 at C/50 (one Na + exchanged in 50 h) until a given voltage (3.07 V and 4.0 V vs. Na/Na + for O1-Na 1 RuO 3 and O1′-Na 1/2 RuO 3 , respectively). The recovered materials were then washed 3 to 5 times with dimethyl carbonate in the glovebox before sending to the synchrotron facility. In situ X-ray diffraction. In situ XRD was carried out in operando using an in situ cell purchased from Bruker on a Bruker-AXS D8 ADVANCE (Co K α radiation) in 0.02 o steps over the 2 θ range of 17–25 o at a C/10 rate. The cell configuration is similar to the one described above except for the positive electrode that consisted in a mixture of Na 2 RuO 3 (85 wt%), acetylene black (10 wt%), and polytetrafluoroethylene (5 wt%). Two layers of glass fiber separators were used to prevent dendrite formation.